Hydrodefluorination of carbon–fluorine bonds by the synergistic action of a ruthenium–palladium catalyst Catalytic hydrodefluorination of organic molecules is a major organometallic challenge, owing to the strength of C–F sigma bonds, and it is a process with multiple industrial applications. Here we report a new heterodimetallic ruthenium–palladium complex based on a triazolyl-di-ylidene ligand. The complex is remarkably active in the hydrodefluorination of aromatic and aliphatic carbon–fluorine bonds under mild reaction conditions. We observe that both metals are required to promote the reaction process. The overall process implies that the palladium fragment facilitates the C–F activation, whereas the ruthenium centre allows the reduction of the substrate via transfer hydrogenation from isopropanol/sodium t -butoxide. The activity of this heterodimetallic complex is higher than that shown by a mixture of the related homodimetallic complexes of ruthenium and palladium, demonstrating the catalytic benefits of the heterodimetallic complex linked by a single-frame ligand. Owing to the high industrial demand of organic molecules that contain carbon–fluorine bonds [1] , [2] , [3] , both C–F bond formation and selective C–F bond activation have become subjects of active investigation [4] , [5] , [6] . Carbon–fluorine bonds are considered as the most passive organic functionalities [7] , [8] , [9] , and their selective activation under mild conditions remains poorly achieved. Although there has been considerable progress in the stoichiometric activation of C–F bonds, the metal-catalysed versions of the process remain relatively scarce [5] , [10] , [11] , [12] , [13] , [14] , [15] , [16] , [17] , [18] , [19] , [20] , [21] . The simplest modification of the C–F bond is its transformation to the simple C–H bond (hydrodefluorination, HDF), a process that has been mainly limited to fluoroarenes, with very few examples referring to trifluoromethylarenes and other perfluoroalkyl groups [1] , [22] , [23] , [24] , [25] , [26] . HDF is an interesting process not only because of the fundamental importance on the C–F bond activation chemistry involved but also because of the potential applications in the activation and disposal of the chlorofluorocarbons, considered as ‘super greenhouse gases’ [27] , [28] , [29] , [30] , [31] . Metal hydrido complexes are often chosen for HDF, but C–F activation can produce stable fluoride complexes, which may hamper catalytic turnover [4] , [15] . Consistent with the decreasing metal–fluoride bond energies, electron-rich metal centres are preferred, but still strong reductants such as high-pressure H 2 or silanes are needed to promote effective HDF, thus often producing over-reduced products. For C 6 F 6− n H n substrates, it has been demonstrated that the C–F bond dissociation energies show a general increase with larger n [32] ; therefore, although the research on the activation of highly fluorinated arenes is mainly focused on selectivity, the search for catalysts that activate low fluorinated arenes is focused on finding effective catalysts that show high activity under the mildest reaction conditions. During the last few years, we have reported efficient methods for the preparation of homo- and heterodimetallic complexes based on a 1,2,4-triazolyl-3,5-di-ylidene ligand, with metals of the platinum group including gold ( Fig. 1 ) [33] , [34] , [35] , [36] , [37] , [38] , [39] . The preparation of such types of heterodimetallic complexes allowed us to study several catalytic processes in which each metal fragment facilitated a mechanistically different cycle [33] , [35] , [36] , [40] . We also confirmed that the presence of the two different metals furnish catalytic benefits compared with the cases in which mixtures of homodimetallic species are used. Exploiting our experience in the preparation of Pd-based catalysts for arene-halogen activation, and Ru-based catalysts for borrowing-hydrogen reactions, here we combine these two metals into one catalyst and explore its performance in the more challenging HDF of fluoroarenes and trifluoromethylarenes. 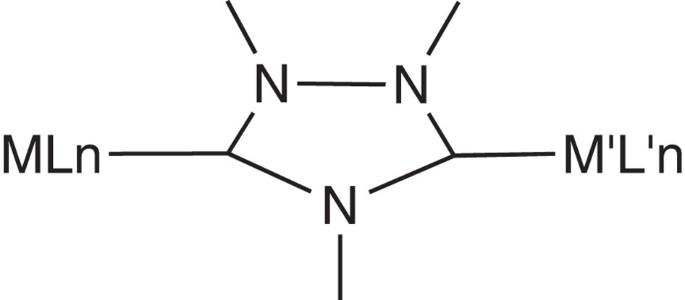Figure 1: Complex formation by the triazolyl-di-ylidene ligand. Schematic representation of homo- and heterodimetallic complexes attached by the triazolyl-di-ylidene ligand. Figure 1: Complex formation by the triazolyl-di-ylidene ligand. Schematic representation of homo- and heterodimetallic complexes attached by the triazolyl-di-ylidene ligand. Full size image 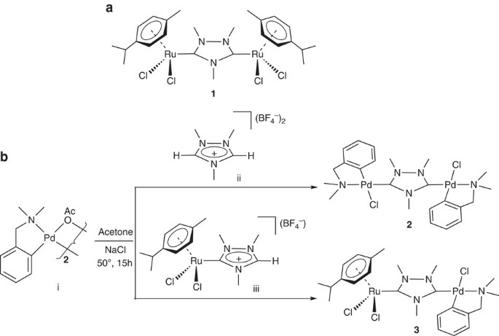Figure 2: Catalysts used in this work. (a) Structure of previously reported complex1. (b) Schematic protocol for the preparation of2and3. Description of the catalysts used Figure 2 shows the complexes under study in this work. All three complexes were obtained from 1,2,4-trimethyl-triazolium tetrafluoroborate, following similar synthetic procedures as those that we have previously reported [33] , [34] , [35] , [36] , [37] , [38] , [39] . The preparation of the Pd-Ru heterodimetallic complex 3 was achieved by the stepwise deprotonation of the triazolium salt, followed by the subsequent addition of the corresponding metal source, as schematically shown in Fig. 2 (below). The preparation of the homodimetallic complex of ruthenium 1 was recently described by us [41] . Complexes 2 and 3 were fully characterized by NMR, high-resolution mass spectroscopy (HRMS) and elemental analysis. Figure 2: Catalysts used in this work. ( a ) Structure of previously reported complex 1 . ( b ) Schematic protocol for the preparation of 2 and 3 . Full size image Catalytic dehalogenation of aryl halides To explore the catalytic activities of 1 – 3 , we first decided to test the three complexes in the dehalogenation of several phenyl halides ( Table 1 ). The reactions were performed in 2-propanol in the presence of t BuONa at 80 °C with a catalyst loading of 1 mol%. In the optimization of the reaction conditions ( Supplementary Table S1 ), we observed that the best results were obtained when carrying out the reactions in the presence of t BuONa, although weaker bases such as Cs 2 CO 3 were also effective. We also carried out the reactions in the absence of catalysts (entries 1, 5 and 9) and observed that all the starting substrate was recovered, indicating that a nucleophilic aromatic substitution does not occur under these reaction conditions. As expected, the bis-ruthenium complex 1 is completely ineffective in the dehalogenation of any of the substrates used. The bis-palladium complex 2 , is capable of moderately dehalogenating bromobenzene (entry 3) and chlorobenzene (entry 7), but is completely ineffective in the HDF of fluorobenzene (entry 11). The heterodimetallic complex 3 is very active in the hydrodehalogenation of all three phenyl halides, affording quantitative conversions to benzene (entries 4, 8 and 12). Interestingly, equimolecular mixtures of 1 and 2 afforded moderate yields of benzene coming from the HDF of fluorobenzene (entry 13), therefore suggesting that the two different metals have a role in the overall process, but also that the presence of these two metals in a single catalyst provides a significant benefit (compare entries 12 and 13). To prove that the reaction is homogeneously catalysed, we also carried out the HDF of fluorobenzene using 3 , in the presence of a mercury drop [42] , and observed that the activity of the catalyst did not change. Although we are aware that the Hg(0) may occasionally lead to inconclusive results [43] , we believe that this experiment supports the idea that the process is homogeneous. Table 1 Catalytic dehalogenation of phenyl halides using catalyst 1– 3 *. Full size table HDF of fluoroarenes To survey the generality and scope of the heterodimetallic Ru/Pd complex, a variety of fluoroarenes was examined ( Table 2 ). As can be seen from the results shown, the Ru/Pd catalyst 3 is highly active in the HDF of a series of arenes with different functional groups, affording good to excellent yields. As we did observe before, the heterodimetallic catalyst 3 always provides the best activities when compared with mixtures of the homodimetallic complexes 1 and 2 (compare entries 1–16). These results suggest that some catalytic cooperativity between the two metals maybe having a role in the catalytic cycle, and that we may have an example of a synergistic effect between ruthenium and palladium. Aryl fluorides possessing electron-withdrawing or electron-donating substituents show very small differences in activity, suggesting that the rate-determining step is not the oxidative addition of the aryl fluoride, as it has been previously observed in the dehalogenation of aryl chlorides [44] , [45] , [46] . Steric factors seem to have an important role, as hindered substrates displayed lower reaction rates, as seen by the lower activities shown by o- fluorotoluene compared with the m - and p -isomers (compare entries 7, 21 and 22). Under the reaction conditions used, the substrates containing carbonyl groups are quantitatively reduced to the corresponding alcohols as a consequence of the catalytic hydrogen transfer from isopropyl alcohol. The HDF of polyfluorinated arenes is exemplified by the reactions of p - and o -difluorobenzene, and 1,3,5-trifluorobenzene, all of which afford benzene in quantitative yields (entries 24–26). Catalyst 3 is also active at a catalyst loading of 0.1 mol%, showing turnover number (TON) values as high as 660 for the HDF of fluorobenzene ( Supplementary Table S2 ), although after 5 h of reaction the reaction was not completed (66%). At this point, it is important to mention that a very small number of examples have been reported in which HDF of fluoroarenes has been carried out using isopropyl alcohol or other secondary alcohols in basic conditions [47] , [48] , [49] , [50] (most of them refer to heterogenous catalysed processes), but as far as we are aware, the heterodimetallic complex 3 seems to be the most active reported to date. Table 2 Hydrodefluorination of fluoroarenes using the complexes 1– 3 *. Full size table The monitoring of the HDF of fluorobenzene by 19 F NMR ( Fig. 3 ) clearly illustrates the different behaviour of the four catalytic systems used for this reaction ( 1 – 3 and 1 + 2 ). The graphic shows that both 3 and a mixture of 1 + 2 are effective in this reaction and that the heterodimetallic catalyst 3 is the most active one. Interestingly, a mixture of the two homodimetallic catalysts 1 and 2 afford almost quantitative conversions after 4 h of reaction, therefore implying that the activity seems to be maintained along all the reaction profile. This result contrasts with the negligible conversions shown by the independent use of 1 and 2 . We believe that these results confirm that only the combination of the palladium and ruthenium fragments result in an effective catalytic system for the HDF reaction of fluorobenzene in the reaction conditions that we used. 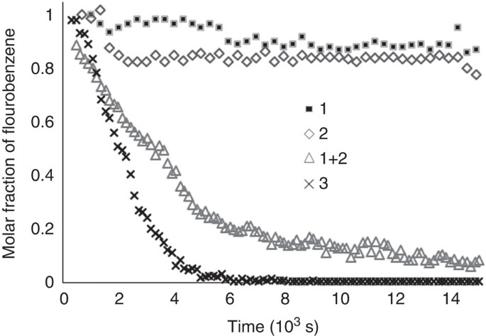Figure 3: Reaction profile of the conversion of fluorobenzene. Reaction conditions: 0.3 mmol of fluoroarene,tBuONa (0.3 mmol), catalyst (1 mol% for1–3, 0.5 mol% of1and 0.5 mol% of2for the mixture1+2), 1.5 ml of 2-propanol at 80 °C. Evolution monitored by19F NMR by measuring the disappearance of the19F resonance of fluorobenzene. Figure 3: Reaction profile of the conversion of fluorobenzene. Reaction conditions: 0.3 mmol of fluoroarene, t BuONa (0.3 mmol), catalyst (1 mol% for 1 – 3 , 0.5 mol% of 1 and 0.5 mol% of 2 for the mixture 1 + 2 ), 1.5 ml of 2-propanol at 80 °C. Evolution monitored by 19 F NMR by measuring the disappearance of the 19 F resonance of fluorobenzene. Full size image To shed some light into mechanistic aspects of the reaction, we carried out the HDF of fluorobenzene and p -fluorotoluene using deuterium-labelled isopropyl alcohol, (CD 3 ) 2 CDOD ( Supplementary Figs S1–S4 ). The characterization of the products resulting from these reactions confirmed the substitution of the fluoride by deuterium, therefore confirming that deuterated isopropyl alcohol is the hydrogen source of the process by transfer hydrogenation. This experiment also allowed us to determine the kinetic isotopic effect ( k H / k D ) by calculating the kinetic constants of the HDF of 4-fluorotoluene and fluorobenzene carried out in isopropyl alcohol and (CD 3 ) 2 CDOD at 80 °C (see Supplementary Figs S1–S4 , and Supplementary Table S3 ). The resulting kinetic isotopic effect values of 2.7 (4-fluorotoluene) and 2.4 (fluorobenzene) suggest that the rate-determining step of the overall process is associated with the reductive part of the reaction, rather than to C–F bond activation. HDF of aliphatic C–F bonds Encouraged by these results, we decided to test catalyst 3 in the HDF of α,α,α-trifluorotoluenes. It is well recognized that these substrates are among the most inert organofluorine compounds, and the reduction of benzylic C–F bonds has not been described until recently [51] . Most of the active catalytic systems used so far refer to early transition metals [22] , [26] and silylium compounds [1] , [24] , [51] , although a few examples also describe the use of late transition metals such as Ru [25] and Ni [52] . As shown in Table 3 , catalyst 3 is capable to HDF a series of trifluorotoluenes in good to excellent yields. The catalyst is very active in the HDF of α,α,α-trifluoro-1-methylnaphthalene, α,α,α-trifluoro-4-methyl-acetophenone and 4-trifluoro-methyl-pyridine (entries 3–6), but provided moderate yields in the HDF of α,α,α-trifluorotoluene, hexafluoro- m -xylene and hexafluoro- p -xylene (entries 1, 9 and 10, respectively). In the case of the hexafluoroxylenes, it is interesting that the reactions selectively yield the HDF of one of the trifluoromethyl groups, whereas the second group remains practically untouched (only traces of the complete dehydrofluorinated compound were detected), regardless of the amount of base used. As we wanted to explore the reasons for the incomplete HDF of these two hexafluoroxylenes, we also performed the reactions with trifluoro- p -xylene, and trifluoro- m -xylene, and observed that the catalyst was ineffective (entries 7 and 8), suggesting that the selective formation of the trifluoroxylenes from the starting hexafluoroxylenes was due to the inert character of the trifluorinated products, rather than to the deactivation of the catalyst during the reaction course. These results are in line with the higher activities shown by trifluorotoluenes with electron-attracting groups, whereas those having electron-donating functionalities are deactivated towards the HDF. It is important to mention that we did not find any reaction intermediates because of the partial HDF of the trifluoromethyl groups, even in reactions with incomplete conversion. Table 3 Hydrodefluorination of trifluorotoluenes with catalyst 3 *. Full size table An interesting result that probably needs a more detailed explanation is the one resulting from the reduction of 4-fluoro-benzotrifluoride ( Table 3 , entry 2), which is reduced to two different products in the presence of four equivalents of base. In this reaction, the reduction of the aromatic C–F bond occurs first, and then the activation of the CF 3 group is produced slowly. In the presence of a lower amount of base (one equivalent), the same substrate undergoes full conversion to trifluorotoluene, therefore implying that only the aromatic C–F bond was reduced, whereas the CF 3 group remained untouched ( Table 2 , entry 20). The selective activation of the aromatic C–F bond in this latter case is obviously because of the amount of base used, and illustrates how the outcome of the process maybe selective to the reduction of aromatic C–F bonds if stoichiometric amounts of base are utilized. All our results indicate that the application of our heterodimetallic catalyst 3 behaves as an effective two-component activation system, which produces significant benefits in the HDF of a wide set of fluorinated organic molecules. The palladium centre would be facilitating the C–F bond activation, while the ruthenium fragment completes the reaction by hydrogenating the substrate. Although a mixture of two different homodimetallic complexes of palladium and ruthenium seem to partially facilitate the process, the reaction is clearly benefited when the two different metal fragments are linked to a single-frame ligand. From a mechanistic point of view, it is difficult to explain the intimate process, which will need a more detailed study, but we believe that we have enough evidence to justify that the most plausible mechanism implies that the action of the two different metals are combined to afford the full HDF reaction. In summary, we have demonstrated the catalytic activity of a heterodimetallic triazolyl-di-ylidene-based ruthenium–palladium complex in the HDF of fluoroarenes and trifluorotoluenes. The catalyst is very efficient in a wide set of substrates, affording quantitative yields for most fluoroarenes in short reaction times (1–2 h) and mild reaction conditions (isopropyl alcohol, 80 °C). We demonstrated that the presence of the two metals is necessary to promote the reaction process, and that the catalytic efficiency is increased when the two metal fragments are bound by a single ligand. These results suggest that some catalytic cooperativity between the two metals should have a role during the catalytic cycle. Although we have already reported several examples of triazolyl-di-ylidene-based heterodimetallic complexes in which each metal promotes a mechanistically distinct process, all the examples that we described until now refer to sequences of independent reactions that are combined into a sophisticated tandem process. This new example is different, in the sense that the two different actions of the metals are combined to afford only one reaction, the hydro(Ru)defluor(Pd)ination, which may not be possible by the action of only one of the metals. General All manipulations were carried out under nitrogen using standard Schlenk techniques and high vacuum, unless otherwise stated. Compounds i [53] , ii [37] , iii [38] and complex 1 [53] were prepared according to the literature procedures. Anhydrous solvents were dried using a solvent purification system (M BRAUN) or purchased from Aldrich and degassed before use by purging with dry nitrogen and kept over molecular sieves. All other reagents were used as received from commercial suppliers. The products were identified by GCMS-QP2010 (Shimadzu) gas chromatograph/mass spectrometer equipped with a Teknokroma (TRB-5MS, 30 m × 0.25 mm × 0.25 μm) column, and the spectra obtained were compared with the standard spectra. The yields, conversion and product selectivity were determined by a GC-2010 (Shimadzu) gas chromatograph equipped with a flame ionization detector and a Teknokroma (TRB-5MS, 30 m × 0.25 mm × 0.25 μm) column. NMR spectra were recorded on Varian Innova spectrometers operating at 300 or 500 MHz ( 1 H NMR) and 75 and 125 MHz ( 13 C NMR), respectively, using CDCl 3 as the solvent at room temperature unless otherwise stated. Elemental analyses were carried out in an EA 1108 CHNS-O Carlo Erba analyser. Electrospray mass spectra were recorded on a Micromass Quatro LC instrument, and nitrogen was employed as drying and nebulizing gas. For HRMS A QTOF I (quadrupole-hexapole-TOF), a mass spectrometer with an orthogonal Z-spray-electrospray interface (Micromass, Manchester, UK) was used. Synthesis of compound 2 Compound ii (48 mg, 0.167 mmol), i (100 mg, 0.167 mmol) and NaCl (50 mg, 0.85 mmol) were refluxed under nitrogen in acetonitrile (10 ml) for 15 h. The final suspension was filtered through Celite and the solvent was evaporated under reduced pressure. Crystallization from dichloromethane/hexane gave pure compound 2 as an off-white crystalline solid. Yield: 90 mg (82%). 1 H NMR (300 MHz, CDCl 3 , Supplementary Fig. S5 ): δ 7.10–6.91 (m, 8H, CH Ar ), 6.90–6.75 (m, 4H, CH Ar ), 6.28 (d, J =7.0 Hz, 2H, CH Ar ), 6.19 (d, J =7.3 Hz, 2H, CH Ar ), 4.36 (s, 6H, N triazole CH 3 ), 4.33 (s, 6H, N triazole CH 3 ), 4.26 (s, 3H, N triazole CH 3 ), 4.23 (s, 3H, N triazole CH 3 ), 4.05–3.88 (m, 8H, N amine CH 2 ), 2.90–2.79 (m, 24H, N amine CH 3 ). 13 C{ 1 H} NMR (75 MHz, CDCl 3 , Supplementary Fig. S6 ): δ 182.6 (C carbene –Pd), 182.4 (C carbene –Pd), (148.4, 147.9, 147.2, 135.8, 134.7, 126.6, 125.9, 124.6, 122.8, 122.5 (C Ar )), (72.5, 72.4 (N amine CH 2 )), (50.6, 50.5, 50.4 (N amine CH 3 )), (41.4, 41.3, 37.7, 37.6 (N triazole CH 3 )). Anal. calcd. for C 23 H 33 N 5 Cl 2 Pd 2 ·3H 2 O (717,34): C, 38,51; H, 5.48; N, 9.76. Found: C, 38.6; H, 5.86; N, 9.67. Electrospray Ms. (Cone 20 V) ( m / z , fragment): 669.0 [M–Cl+ MeCN] + , 337.7 [M–2Cl+ 2MeCN] 2+ . HRMS ESI-TOF-MS (positive mode): [M–Cl+ MeCN] + monoisotopic peak 669.0758; calc. 669.0769, ε r : 1.5 p.p.m. ( Supplementary Fig. S7 ). Synthesis of compound 3 Compound iii (100 mg, 0.198 mmol), i (59 mg, 0.099 mmol) and NaCl (79 mg, 1.35 mmol) were stirred under nitrogen in deoxygenated acetone (10 ml) at 50 °C for 15 h. The final suspension was filtered through Celite and the solvent was removed under reduced pressure. The crude solid was purified by column chromatography. Elution with a mixture of CH 2 Cl 2 /acetone (4:6) afforded an orange band. Crystallization from dichloromethane/hexane gave compound 2 as an orange crystalline solid. Yield: 100 mg (73%). 1 H NMR (300 MHz, CDCl 3 , Supplementary Fig. S8 ): δ 6.96 (m, 2H, CH Ar ), 6.78 (m, 1H, CH Ar ), 6.24 (d, 3 J H,H =7.5 Hz, 1H, CH Ar ), 5.56 (d, 3 J H,H =6.0 Hz, 1H, CH p- cym ), 5.53 (d, 3 J H,H =5.8 Hz, 1H, CH p- cym ), 5.31 (d, 3 J H,H =5.9 Hz, 1H, CH p- cym ), 5.18 (d, 3 J H,H =5.9 Hz, 1H, CH p- cym ), 4.41 (s, 3H, N triazole CH 3 ), 4.35 (s, 3H, N triazole CH 3 ), 4.30 (s, 3H, N triazole CH 3 ), 3.93 (dd, 3 J H,H =45.3, 14.0 Hz, 2H, N amine CH 2 ), 2.99 (sept, 3 J H,H =6.9 Hz, 1H, CH isop p- cym ), 2.85 (s, 3H, N amine CH 3 ), 2.83 (s, 3H, N amine CH 3 ), 2.13 (s, 3H, CH 3 p -cym ), 1.33 (d, 3 J H,H =4.1 Hz, 3H, CH 3isop p -cym ), 1.31 (d, 3 J H,H =4.1 Hz, 3H, CH 3isop p -cym ). 13 C{ 1 H} NMR (75 MHz, CDCl 3 , Supplementary Fig. S9 ): δ 186.4 (C carbene –Ru), 182.4 (C carbene –Pd), (147.8, 146.9, 136.1, 126.5, 124.6, 122.4 (C Ar )), (110.2, 99.4 (Cq p -cym )), (87.3, 86.3, 84.2, 82.9 (CH p -cym )), 72.3 (N amine CH 2 ), (50.7, 50.4 (N amine CH 3 )), (42.2, 38.5, 37.9 (N triazole CH 3 )), 30.8 (CH isop p- cym ), (22.6, 22.3 (CH 3isop p- cym )), 18.8 (CH 3 p- cym ). Anal. calcd. for C 24 H 35 N 4 Cl 3 RuPd·2H 2 O (729.44): C, 39.51; H, 5.38; N, 7.68. Found: C, 40.0; H, 5.77; N, 7.75. Electrospray Ms. (Cone 20 V) ( m / z , fragment): 700.1 [M–Cl+ MeCN] + .HRMS ESI-TOF-MS (positive mode): [M–Cl] + monoisotopic peak 659.0305; calc. 659.0319, ε r : 2.1 p.p.m. ( Supplementary Fig. S10 ). HDF of fluoroarene compounds The catalyst (1 mol%) and tBuONa (0.3 mmol) were placed together in a thick-walled Schlenk tube with a Teflon cap. The tube was then evacuated and filled with nitrogen three times. 2-propanol (2 ml) and fluoroarene (0.3 mmol) were added and the mixture was stirred at 80 °C for the desired time. Yields were determined by gas chromatography analyses using anisole (0.3 mmol) as an internal standard. Isolated products were characterized by 1 H NMR and 13 C NMR after extraction with dichloromethane and a saturated NaCl solution (3 × 5 ml). HDF of fluoroalkyl compounds The heterodimetallic complex 3 (5 mol%) and tBuONa (0.9 mmol) were placed together in a thick-walled Schlenk tube with a Teflon cap. The tube was then evacuated and filled with nitrogen three times. 2-propanol (2 ml) and fluoroalkyl (0.3 mmol) were added and the mixture was stirred at 80 °C for the desired time. Yields were determined by gas chromatography analyses using anisole (0.3 mmol) as the internal standard. Isolated products were characterized by 1 H and 13 C NMR after extraction with dichloromethane and a saturated NaCl solution (3 × 5 ml). Kinetic measurements A J. Young tube was loaded with catalyst 3 (1 mol%) and tBuONa (0.3 mmol). The tube was then evacuated and filled with nitrogen three times. 2-propanol (1 ml) and fluoroarene (0.3 mmol) were added and the mixture was stirred at room temperature until homogeneous solution was formed. The tube was then introduced in an NMR probe preheated at 80 °C. The conversion of fluoroaromatic compound was monitored by 19 F NMR spectroscopy at intervals over the course of the desired time. The corresponding deuterated products were identified by GCMS-QP2010, 1 H NMR and 13 C NMR. How to cite this article: Sabater, S. et al. Hydrodefluorination of carbon–fluorine bonds by the synergistic action of a ruthenium–palladium catalyst. Nat. Commun. 4:2553 doi: 10.1038/ncomms3553 (2013).